Phosphoric acid-catalyzed atroposelective construction of axially chiral arylpyrroles Axially chiral arylpyrroles are key components of pharmaceuticals and natural products as well as chiral catalysts and ligands for asymmetric transformations. However, the catalytic enantioselective construction of optically active arylpyrroles remains a formidable challenge. Here we disclose a highly efficient strategy to access enantioenriched axially chiral arylpyrroles by means of organocatalytic atroposelective desymmetrization and kinetic resolution. Depending on the remote control of chiral catalyst, the arylpyrroles were obtained in high yields and excellent enantioselectivities under mild reaction conditions. This strategy tolerates a wide range of functional groups, providing a facile avenue to approach axially chiral arylpyrroles from simple and readily available starting materials. Selected arylpyrrole products proved to be efficient chiral ligands in asymmetric catalysis and also important precursors for further synthetic transformations into highly functionalized pyrroles with potential bioactivity, especially the axially chiral fully substituted arylpyrroles. Axially chiral arylpyrroles constitute the core skeletons of a wide range of natural products [1] , [2] , [3] and pharmaceutical agents [4] , [5] , [6] . Owing to their intrinsic structure characteristics, they proved to possess widespread applications in organic synthesis [7] , [8] , [9] , [10] , [11] , [12] , [13] , [14] , [15] . For example, arylpyrroles scaffolds occur in plenty of chiral phosphine ligands applied in numerous transition metal-mediated reactions (Fig. 1 ) [7] , [8] , [9] . More importantly, the optically pure arylpyrrole derivatives have been extensively used in current asymmetric reactions [10] , [11] , [12] , [13] , [14] as chiral resolving agents [10] , [11] , chiral ligands [12] , [13] as well as chiral catalysts [14] . Nonetheless, over the past decade, conventional approaches to access these optically active arylpyrroles were by optical resolution of the racemates using chiral resolution agents or chiral column chromatography, which not only required the stoichiometric amounts of chiral reagent, but also were limited by the substrate scope [10] , [15] , [16] . While the first catalytic asymmetric Paal–Knorr reaction was established to access highly enantioenriched axially chiral arylpyrroles by our group recently [17] , complicated catalytic system and narrow substrate range restricted its application. Therefore, the atroposelective construction of axially chiral arylpyrroles remains comparatively unexplored and the development of facile and direct route is highly appealing. Fig. 1 Representative molecules containing axially chiral arylpyrrole frameworks. a Bioactive natural products. b Resolving agent. c Chiral ligands and catalysts Full size image Recently, Bencivenni’s group reported a pioneering study on the remote control of the axial chirality of atropisomeric succinimides through vinylogous Michael addition reaction via aminocatalytic desymmetrization of arylmaleimides (Fig. 2a ) [18] , [19] , [20] . The key feature of this method relies on the recognition of the catalyst with regards to the maleimide’s symmetry plane. The hydrogen bonding between the oxygen of the carbonyl group of the substrate and the protonated quinuclidine moiety of the catalyst is crucial for the excellent stereoselectivity. Inspired by this elegant work involving the remote control of the axial chirality, as well as our ongoing interest in chiral phosphoric acid (CPA) catalytic atroposelective synthesis of enantioenriched axially chiral structures [21] , [22] , we envisage that the readily available 2,5-disubstituted arylpyrroles should be suitable prochiral substrates to afford the expected axially chiral structures by enantioselective desymmetrization [23] , [24] , [25] , [26] or kinetic resolution [27] , [28] , [29] , [30] , [31] , [32] under the strategy of remote stereocontrol by organocatalysts (Fig. 2b ) [33] , [34] , [35] , [36] . However, the major challenges in this scenario would be: (1) the choice of appropriate electrophilic reagents could react efficiently with the arylpyrroles. Meanwhile, the electrophiles would interact with the organocatalyst in a reasonable spatial configuration to enhance the reactivity and offer an ideal chiral environment for the control of the atroposelectivity; (2) the careful selection of compatible chiral organocatalyst to effectively induce the axial chirality since the distance between the chiral axis and the catalyst activation site is relatively long; (3) lacking an available proton donor group on the arylpyrroles for hydrogen bonding effect, the interaction between arylpyrrole substrates and the chiral catalyst could not occur effectively [37] , [38] , [39] , [40] , [41] , [42] , [43] , [44] . Herein, we present our strategy to overcome the abovementioned challenges and successfully construct the highly enantioenriched axially chiral arylpyrroles by means of the remote control of the axial chirality. Two complementary approaches, namely desymmetrization/kinetic resolution, are devised with CPA as the catalyst to give the axially chiral arylpyrroles with highly structural diversity and excellent enantiocontrol. These optical active axially chiral arylpyrroles are able to sever as chiral building blocks for rapid transformations to functionalized pyrroles with potential bioactivity and ligands for asymmetric catalytic reactions. Fig. 2 Background and project synopsis. a Aminocatalytic enantioselective synthesis of atropisomeric succinimides via remote control strategy (Bencivenni’s work). b Our strategy for the remote enantiocontrol of axially chiral arylpyrroles. Black circle, sterically bulky substituent Full size image Reaction condition optimization To validate the feasibility of the hypothesis, the reaction of 1-(2-( tert -butyl)phenyl)-2,5-dimethyl-1 H -pyrrole 1a and diethyl ketomalonate 2a were conducted with 10 mol% SPINOL-derived CPA ( S )- C1 in toluene at room temperature. 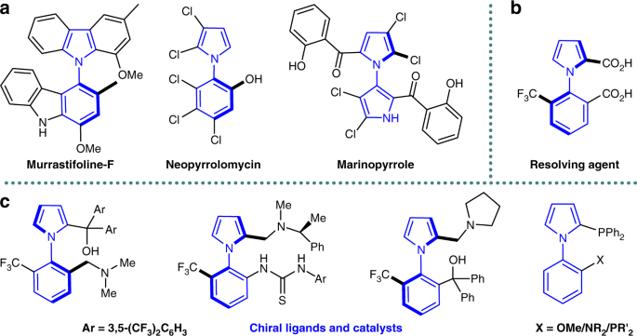Fig. 1 Representative molecules containing axially chiral arylpyrrole frameworks.aBioactive natural products.bResolving agent.cChiral ligands and catalysts Encouragingly, the reaction proceeded smoothly to give the desired axially chiral arylpyrrole 3a in 74% yield (Table 1 , entry 1). Despite only 22% ee, this result clearly demonstrated that the organocatalytic remote control of the chiral axis of arylpyrroles by desymmetrization strategy was feasible. To improve reaction outcomes, we turned our attention to explore the effect of the catalysts. As shown in Table 1 , all the tested CPAs were capable of catalyzing this reaction to give 3a in reasonable to excellent yields (Table 1 , entries 2–8). These results also evidenced that CPAs containing bulky substituents could significantly enhance the stereocontrol of the reaction and H 8 -BINOL-derived ( S )- C8 with 2,4,6-triisopropylphenyl group on the 3,3′-position was superior to other catalysts to give the desired product 3a in 93% yield with 90% ee. After that, various solvents were evaluated to prove the cyclohexane as the optimal reaction solvent (Table 1 , entries 8–12). Lower reaction temperature resulted in negligible effect in enantioselectivity, accompanied by the loss of chemical yield (Table 1 , entry 13). Further optimization revealed that 5 mol% catalyst loading could uphold the enantioselectivity effectively with slight increase of chemical yield when the reaction time was extended to 36 h (Table 1 , entries 14 and 15). Based on the above results (See Supplementary Tables 1 –4), the optimized conditions were concluded as follows: treatment of 2a with 1.5 equivalent of 1a in cyclohexane at room temperature in the presence of 5 mol% of ( S )- C8 and the reaction could give the desired axially chiral arylpyrrole 3a in 96% isolated yield with 95% ee (Table 1 , entry 15). Table 1 Optimization of reaction conditions. a Full size table Substrate scope After establishing the optimal reaction conditions, we set out to explore the substrate generality of this transformation. Firstly, the substrate scope with respect to the symmetrical arylpyrroles was investigated ( 1a – 1r ). 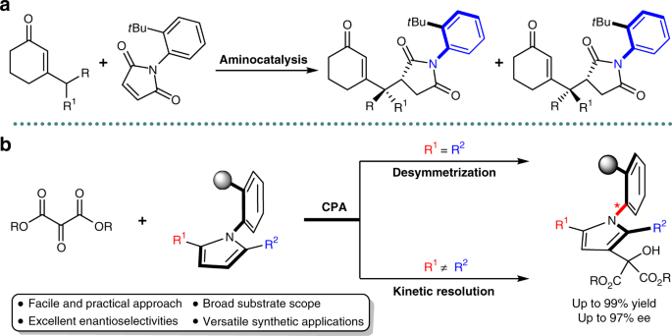Fig. 2 Background and project synopsis.aAminocatalytic enantioselective synthesis of atropisomeric succinimides via remote control strategy (Bencivenni’s work).bOur strategy for the remote enantiocontrol of axially chiral arylpyrroles. Black circle, sterically bulky substituent Most reactions could be completed within 64 h to give the desired axially chiral arylpyrroles (Table 2 , 3a – 3r ) in high yields (82–99%) with excellent enantioselectivities (83–97% ee). It is noteworthy to point out that the ortho group on the phenyl ring is not only restricted to t butyl group, iodo, isopropyl, trifluoromethyl, diphenyl phosphine, 2-isopropenyl, styrene as well as cyclohexene groups were also applicable to give the expected products with good to excellent enantiocontrol ( 3g – 3q ). Subsequently, symmetrical arylpyrroles 1r bearing diethyl group could afford 3r in excellent yield and good enantioselectivity. Moreover, varying the ester moiety of ketomalonate could also result in excellent enantioselectivities ( 3s– 3u ). Notably, 1o with a diphenyl phosphine substituent was converted to the corresponding product 3o and 3 u as potential chiral phosphine ligands. Besides, the halide substituents in the obtained arylpyrroles provided opportunities for the downstream coupling reactions to set up a compound library by routine transition metal-catalyzed reactions. Furthermore, the absolute configurations of the axially chiral products were assigned to be ( aR ) by X-ray crystallographic analysis of 3 s and those of the other products were assigned by analogy (see Supplementary Figure 1). To verify the practicality of such method, a gram-scale reaction was carried out for the synthesis of 3a under the optimal reaction conditions. As displayed in Table 2 , no significant variation was detected in terms of the chemical yield and stereoselectivity as compared to the small scale reaction. Table 2 Substrate scope with respect to symmetric prochiral arylpyrroles. 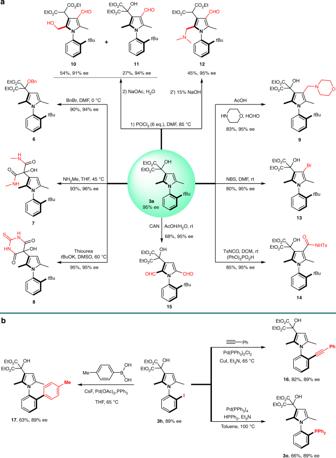Fig. 3 Versatile synthetic transformations.aSynthetic transformations of compound3a. Ts,p-toluenesulfonyl.bSynthetic transformations of compound3h 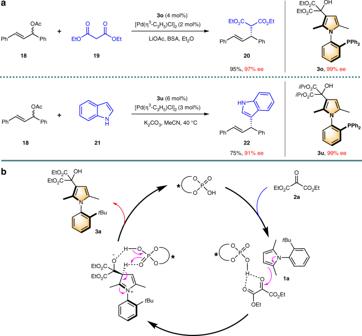Fig. 4 Applications in asymmetric catalysis and plausible mechanism.aAsymmetric catalysis applications.bProposed reaction mechanism a Full size table Table 3 Substrate scope with respect to asymmetric racemic arylpyrroles. a Full size table Encouraged by the above results about the construction of axially chiral arylpyrroles via atroposelective desymmetrization of symmetric substrates, we continued to explore the feasibility of this reaction with asymmetric racemic arylpyrroles by using kinetic resolution to further expand the substrate scope. Plenty of asymmetric arylpyrrole racemates with aromatic substituents on the pyrrole ring were then prepared and subjected to the standard conditions. The results were summarized in Table 3 and all the reactions underwent smoothly to give good to high selectivity factor ( S = 32–69, 5a – 5l ). The corresponding products were obtained in 87–94% ee with 42–47% isolated yields regardless of the steric and electronic properties of the substituents. Notably, substrates possessing a naphthyl or thienyl group ( 5j– 5l ) also worked efficiently to afford high selectivity, respectively. Moreover, replacement of aromatic substitutions with alkyl group gave rise to unobvious effect on the reaction outcomes ( 5m – 5n ). Our method thus represents one of the most straightforward syntheses of axially chiral arylpyrrole and its analogs. The absolute configuration of 5a was attributed to be ( aS ) by X-ray crystallographic analysis and those of the other products were assigned by analogy (see Supplementary Figure 2). Versatile synthetic transformations To demonstrate the synthetic utility of the obtained axially chiral arylpyrroles, a series of chemical transformations were then conducted (Fig. 3a ). Firstly, the free OH group of the axially chiral arylpyrrole 3a could be easily protected by a benzyl group to yield compound 6 . Next, the treatment of compound 3a with thiourea or methylamine gave the corresponding diamide 7 or thiobarbituric structure 8 in almost quantitative yield without any erosion of enantioselectivity [45] , [46] . While highly functionalized pyrroles show a wide spectrum of bioactivities, very few methods are available to access these frameworks [47] , particularly penta-substituted axially chiral arylpyrroles. Gratifying, the fully substituted axially chiral pyrroles 9 , 10 , 11 , and 12 could be generated from 3a by classic Mannich and Vilsmeier–Haack reaction, respectively in moderate yields with highly preserved chiral integrity [48] . Subsequently, bromination of 3a with NBS gave axially chiral arylpyrrole 13 in 80% yield, which could be employed as a precursor to prepare fully substituted axially chiral pyrroles by the following coupling reactions. Furthermore, the treatment of 3a with 4-methyl-benzenesulfonylisocyanate provided compound 14 without loss of stereochemical integrity. Noteworthy, arylpyrrole ( R )- 3a could be readily oxidized to dialdehyde 15 with cerium(IV) ammonium nitrate as the oxidative reagent [49] . Moreover, the obtained product 3 h possessing an iodo substituent was an applicable reactant for classic transition metal-mediated coupling reactions (Fig. 3b ). For instance, the Sonogashira reaction proceeded smoothly to furnish the desired product 16 with a synthetic useful alkynyl group in 82% yield, while compound 17 was produced efficiently by Suzuki coupling with organoboronic acid in the presence of palladium catalyst. Apart from that, the verified axially chiral phosphine ligand 3o could also be synthesized from 3 h via rapid C–P bond formation in 66% yield. Notably, no ee erosion was detected for all these reactions. Fig. 3 Versatile synthetic transformations. a Synthetic transformations of compound 3a . Ts, p -toluenesulfonyl. b Synthetic transformations of compound 3 h Full size image Configurational stability test and catalytic applications The investigation for the configurational stability of the product was conducted by heating a solution of 3a in different solvent ( i PrOH, DCE, and toluene) at up to 150 °C for 24 h. Deteriorations of stereochemical integrity were negligible even under the conditions which the substrate began to decompose. Similar experimental results were obtained with 3o and 5c as the test objects (see Supplementary Table S6–S8). Therefore, this kind of axially chiral compounds displayed a high-rotation energy and may have potential applications as organocatalysts/ligands. Finally, we evaluated the applicability of the resulted axially chiral arylpyrrole in asymmetric catalysis. Compound 3o (99% ee, after semipreparative high-performance liquid chromatography (HPLC) enantioseparation) was then selected as the ligand for the palladium catalyzed allylic alkylation [50] . Gratifyingly, the reaction of racemic 18 and malonate 19 proceeded effectively with 2 mol% of palladium catalyst and 4 mol% of 3o to give the desired product 20 in 95% yield with 97% ee. Aside from 3o , compound 3 u (99% ee, recrystallization with Et 2 O/hexane) could also work well in this type of reaction with indole as the nucleophile, indicating that the resulted highly enantioenriched axially chiral arylpyrrole is capable of inducing the chirality in asymmetric synthesis (Fig. 4a ). Further studies with regard to the application of axially chiral arylpyrroles as catalysts or ligands for asymmetric reactions are currently under active investigations. Fig. 4 Applications in asymmetric catalysis and plausible mechanism. a Asymmetric catalysis applications. b Proposed reaction mechanism Full size image Plausible mechanism A monofunctional activation mode was proposed in Fig. 4b for this asymmetric transformation based on the experimental results and the reports from Terada [51] and Rueping [52] . The hydrogen bonding between ketomalonate and CPA was the pivotal interaction to form the chiral pocket [37] for the induction of chirality. The second carbonyl of the ketomalonate is essential to fix the whole system in a rigid configuration. Besides, such a pathway basically coincides with the plausible mechanism provided by List and Liu et al. for the addition of indolizines and N -methylpyrroles to enones and imines [38] , [39] , [40] . In conclusion, we have successfully developed a highly efficient and practical approach for the atroposelective synthesis of axially chiral arylpyrrole derivatives through two complementary asymmetric transformations (desymmetrization/kinetic resolution). Excellent yields and enantioselectivities were obtained with CPA as the chiral catalyst. The key feature of this approach is the achievement of axial chirality via remote control manner, allowing the chiral catalyst to transfer its stereochemical properties along the C–N axis of arylpyrrole. Moreover, highly enantioenriched arylpyrroles proved to be efficient chiral ligands in asymmetric catalysis and versatile building blocks to access other useful axially chiral molecules. Diversified synthetic transformations demonstrated the utilities of this approach, yielding a variety of functionalized axially chiral arylpyrroles, especially the axially chiral penta-substituted arylpyrroles. General information Chemicals were purchased from commercial suppliers and used without further purification unless otherwise stated. CPA was purchased from Daicel Chiral Technologies (China). Analytical thin layer chromatography (TLC) was performed on precoated silica gel 60 GF254 plates. Flash column chromatography was performed using Tsingdao silica gel (60, particle size 0.040–0.063 mm). Visualization on TLC was achieved by use of UV light (254 nm) or iodine. Nuclear magnetic resonance (NMR) spectra were recorded on a Bruker DPX 400 spectrometer at 400/500 MHz for 1 H NMR, 100/125 MHz for 13 C NMR and 376 MHz for 19 F NMR in CDCl 3 , DMSO-d 6 with tetramethylsilane (TMS) as internal standard. The chemical shifts are expressed in ppm and coupling constants are given in Hz. Data for 1 H NMR are recorded as follows: chemical shift (δ, ppm), multiplicity (s = singlet; d = doublet; t = triplet; q = quartet; p = pentet; m = multiplet; br = broad), coupling constant (Hz), integration. Data for 13 C NMR are reported in terms of chemical shift (δ, ppm). Mass spectrometric data were obtained using Bruker Apex IV RTMS. The enantiomeric excess values were determined by chiral HPLC with an Agilent 1200 LC instrument and CHIRALPAK and CHIRALCEL columns. High resolution mass spectroscopy analyses were performed at a Bruker Daltonics. Inc mass instrument (electrospray ionization (ESI)), Thermo Scientific. Q-Exactive (heated ESI (HESI)), and Thermo Scientific. Orbitrap Fusion (HESI). General procedure for the synthesis of racemic 3 An oven-dried 10 mL of Schlenk tube was charged with arylpyrroles 1 (0.15 mmol), 1 mL of CH 2 Cl 2 and diphenyl phosphate (0.01 mmol) at ambient temperature. Then, ketomalonate 2 (0.10 mmol) was added to the above solution and the mixture was stirred until the starting material was completely consumed. The mixture was concentrated under reduced pressure and purified by flash column chromatography (ethyl acetate/petroleum ether) to afford the corresponding racemic product 3 . General procedure for the synthesis of ( R )- 3 An oven-dried 10 mL of Schlenk tube was charged with arylpyrroles 1 (0.30 mmol), ( S )- C8 (0.01 mmol), 2.0 mL of dry cyclohexane, and the mixture was stirred at ambient temperature for 10 min. A solution of ketomalonate 2a (0.20 mmol) in dry cyclohexane (1.0 mL) was added dropwise to the above solution and the mixture was stirred until the starting material was completely consumed. Then the mixture was concentrated under reduced pressure and purified by flash chromatography eluted with PE/EA (10/1 to 5/1) to afford the corresponding axially chiral arylpyrrole products ( R )- 3 . For 3g– 3i , m , 3r , the reaction conditions are as follows: an oven-dried 10 mL of Schlenk tube was charged with arylpyrroles 1 (0.30 mmol), ( S )- C8 (0.02 mmol) and 1.5 mL of mixed solvent (cyclohexane/methylcyclohexane = 1/1). After the mixture was stirred at −30 °C for 30 min, a solution of ketomalonate 2a (0.20 mmol) in 1.5 mL of mixed solvent (0.75 mL cyclohexane/0.75 mL methylcyclohexane) was added dropwise to the above solution and the mixture was stirred until the starting material was completely consumed. Then the mixture was concentrated under reduced pressure and purified by flash chromatography eluted with PE/EA (10/1 to 5/1) to afford the corresponding axially chiral arylpyrrole products. General procedure for the synthesis of racemic 5 An oven-dried 10 mL of Schlenk tube was charged with arylpyrrole 4 (0.20 mmol), 1 mL cyclohexane and rac - C8 (0.01 mmol) at ambient temperature. Then, ketomalonate 2a (0.10 mmol) was added to the above solution and the mixture was stirred until the starting material was completely consumed. The mixture was concentrated under reduced pressure and purified by flash column chromatography (ethyl acetate/petroleum ether) to afford the corresponding racemic product 5 . Notably, there was also by-product 5′ was obtained, which is the isomer of 5 . General procedure for the kinetic resolution of 4 Under nitrogen atmosphere, an oven-dried 10 mL of Schlenk tube was charged with asymmetric arylpyrroles rac - 4 (0.40 mmol), ( S )- C8 (0.02 mmol), 2.4 mL of dry cyclohexane, and the mixture was stirred at 30 °C for 10 min. Then, a solution of ketomalonate 2a (0.20 mmol) in dry cyclohexane (2.4 mL) was added dropwise to the above solution and the mixture was stirred until the starting material was completely consumed, then the mixture was concentrated under reduced pressure and purified by flash chromatography eluted with PE/EA (10/1 to 5/1) to afford the corresponding axially chiral arylpyrroles product 5 and recovered substrates ( R )- 4 .